Synapsin II desynchronizes neurotransmitter release at inhibitory synapses by interacting with presynaptic calcium channels In the central nervous system, most synapses show a fast mode of neurotransmitter release known as synchronous release followed by a phase of asynchronous release, which extends over tens of milliseconds to seconds. Synapsin II ( SYN2 ) is a member of the multigene synapsin family ( SYN1/2/3 ) of synaptic vesicle phosphoproteins that modulate synaptic transmission and plasticity, and are mutated in epileptic patients. Here we report that inhibitory synapses of the dentate gyrus of Syn II knockout mice display an upregulation of synchronous neurotransmitter release and a concomitant loss of delayed asynchronous release. Syn II promotes γ-aminobutyric acid asynchronous release in a Ca 2+ -dependent manner by a functional interaction with presynaptic Ca 2+ channels, revealing a new role in synaptic transmission for synapsins. Neurotransmitter release is a tightly regulated process that allows neurons to communicate with each other. Most of the fast communication at the synaptic level is based on a synchronous process of neurotransmitter release in response to the action potential. However, the majority of CNS synapses also show an asynchronous component of neurotransmitter release following stimulation [1] , [2] , [3] , [4] , [5] , [6] , [7] . Asynchronous release is not fully time-locked to the presynaptic stimulus, is Ca 2+ -dependent, and is usually enhanced by the residual build-up of Ca 2+ after repetitive stimulation [5] , [7] , [8] . Synaptotagmins, a family of presynaptic Ca 2+ -sensor proteins, have a fundamental role in the control of the synchronous and asynchronous modes of release, with distinct isoforms regulating different components of release [9] , [10] , [11] , [12] . Doc2, another presynaptic Ca 2+ sensor, promotes asynchronous neurotransmitter release at excitatory synapses [13] and VAMP4, a vesicle-associated SNARE protein, maintains asynchronous release at inhibitory synapses [14] . Synapsins (Syn I, II and III) are a family of phosphoproteins that coat synaptic vesicles (SVs) and have important roles in neural development, synaptic transmission and plasticity [15] . The best described function of Syns is the control of neurotransmitter release by clustering SVs and tethering them to the actin cytoskeleton, thus maintaining the integrity of the reserve SV pool [15] , [16] . Moreover, at least in inhibitory synapses, Syns appear to control downstream events of SV exocytosis, such as docking and fusion and, implicitly, the size of the readily releasable pool (RRP) [16] , [17] . Mutant mice lacking one or more Syn isoforms are all prone to epileptic seizures, with the exception of Syn III knockout (KO) mice [15] , [18] . Genetic mapping analysis identified SYN2 among a restricted number of genes significantly contributing to epilepsy predisposition [19] , [20] and mutations in the SYN1 gene have been reported to have a causal role in epilepsy and/or autism [21] , [22] . Synapsin II appears to have a specific role in preventing synaptic depression and maintaining the reserve pool of SV at central excitatory synapses and neuromuscular junction [23] , [24] , [25] , but its role in inhibitory synaptic transmission is not yet understood. Here, we investigated the consequences of Syn II deletion on basal neurotransmitter release and short-term plasticity at hippocampal inhibitory and excitatory synapses. The deletion of Syn II results in an increase of synchronous inhibitory transmission, while the asynchronous component of neurotransmitter release is virtually abolished selectively in inhibitory synapses. Moreover, we show that this action of Syn II is Ca 2+ -dependent and that Syn II interacts directly with presynaptic Ca 2+ channels to modulate the ratio between synchronous and asynchronous GABA (γ-aminobutyric acid) release. Post-docking roles of Syn II at inhibitory synapses We first investigated the functional effects of Syn II deletion on neurotransmitter release at both inhibitory and excitatory synapses. To this purpose, we made whole-cell voltage-clamp recordings of dentate gyrus granule neurons in hippocampal slices of 3-week-old Syn II KO and age-matched WT mice. We employed extracellular stimulation (see Methods) of the medial perforant path to elicit monosynaptic inhibitory [26] ( Supplementary Fig. S1 ) or excitatory ( Supplementary Fig. S2 ) responses in granule cells. While no changes were observed in the evoked excitatory postsynaptic currents ( Supplementary Fig. S2 ), the amplitude of evoked inhibitory postsynaptic currents (eIPSCs) was significantly higher in KO neurons (78.14±7.83 pA; n =36 neurons/17 mice for WT neurons; 120.11±9.85 pA, n =39 neurons/20 mice for KO neurons; P =0.001) ( Fig. 1a ). This increase in amplitude was not accompanied by changes in the total area of the response (4.11±0.39 and 4.24±0.43 pC, for WT and KO neurons, respectively, P =0.52) ( Fig. 1b ), suggesting alterations in the kinetics of release. By fitting the deactivation time-course of the eIPSCs with a biexponential function, we observed that the fast component ( τ fast ) of the response was unchanged between genotypes (10.57±0.72 and 9.75±0.97 ms, for WT and KO neurons, respectively, P =0.49), whereas the slow component ( τ slow ) of the decay was significantly faster in KO neurons (35.29±2.01 and 28.75±1.92 ms, for WT and KO neurons, respectively, P =0.029) ( Fig. 1c ). This effect can explain the apparent inconsistency between the lack of difference in the total charge and the clear increase of the eIPSC amplitude ( Fig. 1b ). 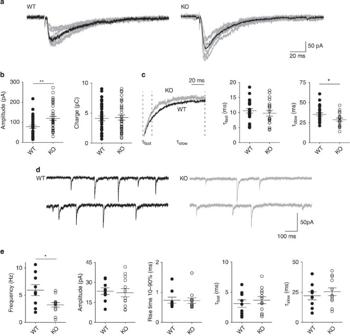Figure 1: Syn II deletion modifies the dynamics of the evoked GABA response. (a) Representative traces of eIPSCs from WT and KO dentate gyrus granule neurons (the average trace is shown in black). (b) Mean (±s.e.m.) amplitude and charge of eIPSCs (closed and open circles represent single experiments for WT and KO neurons, respectively). (c) The decay of the WT eIPSC (left panel; black trace) was normalized to the peak amplitude of the KO eIPSC (grey trace). A two-exponential model was used to fit the fast and slow components of the decay (τfastandτslow) and their average values (±s.e.m.) are shown in the middle and right panels, respectively. *P<0.05, two-tailed unpaired Student’st-test.n=23 andn=30 neurons for WT (10 mice) and KO (15 mice), respectively. Analysis of eIPSC kinetics showed that the latency (2.06±0.19 and 1.78±0.28 ms, for WT and KO neurons, respectively,P=0.45) and rise time (2.74±0.34 and 2.85±0.32 ms, for WT and KO neurons, respectively,P=0.81) were similar between genotypes (data not shown). (d) Representative traces of mIPSCs recorded in dentate gyrus granule neurons from WT (black) and KO (grey) mice. (e) Aligned dot plots of frequency, amplitude and kinetic parameters (rise time;τfast;τslow) of mIPSCs in neurons from WT (closed symbols) and KO (open symbols) mice. Each dot represents one experiment. *P<0.05, two-tailed unpaired Student’st-test.n=9 andn=13 neurons from WT (4 mice) and KO (6 mice), respectively. Figure 1: Syn II deletion modifies the dynamics of the evoked GABA response. ( a ) Representative traces of eIPSCs from WT and KO dentate gyrus granule neurons (the average trace is shown in black). ( b ) Mean (±s.e.m.) amplitude and charge of eIPSCs (closed and open circles represent single experiments for WT and KO neurons, respectively). ( c ) The decay of the WT eIPSC (left panel; black trace) was normalized to the peak amplitude of the KO eIPSC (grey trace). A two-exponential model was used to fit the fast and slow components of the decay ( τ fast and τ slow ) and their average values (±s.e.m.) are shown in the middle and right panels, respectively. * P <0.05, two-tailed unpaired Student’s t -test. n =23 and n =30 neurons for WT (10 mice) and KO (15 mice), respectively. Analysis of eIPSC kinetics showed that the latency (2.06±0.19 and 1.78±0.28 ms, for WT and KO neurons, respectively, P =0.45) and rise time (2.74±0.34 and 2.85±0.32 ms, for WT and KO neurons, respectively, P =0.81) were similar between genotypes (data not shown). ( d ) Representative traces of mIPSCs recorded in dentate gyrus granule neurons from WT (black) and KO (grey) mice. ( e ) Aligned dot plots of frequency, amplitude and kinetic parameters (rise time; τ fast ; τ slow ) of mIPSCs in neurons from WT (closed symbols) and KO (open symbols) mice. Each dot represents one experiment. * P <0.05, two-tailed unpaired Student’s t -test. n =9 and n =13 neurons from WT (4 mice) and KO (6 mice), respectively. Full size image Differences in the amplitude and kinetics of the inhibitory response may have a postsynaptic origin, as changes in the subunit composition of GABA A receptors can influence both parameters [27] . To clarify this matter, we recorded miniature inhibitory postsynaptic currents (mIPSCs) from granule neurons in the presence of 0.3 μM TTX. We noticed a reduction in the frequency of mIPSCs in KO neurons (5.91±1.00 and 3.18±0.42 Hz, for WT and KO neurons, respectively; P =0.011; Fig. 1d ), pointing to a presynaptic defect. Neither amplitude (23.43±2.51 and 22.19±3.04 pA, for WT and KO neurons, respectively, P =0.75) nor kinetics of mIPSCs (rise time 10–90%: 0.73±0.10 and 0.72±0.09 ms, P =0.90; τ fast : 3.09±0.62 and 3.67±0.58 ms, P =0.516; τ slow : 22.01±3.33 and 25.40±3.20 ms, P =0.48; n =9 neurons/4 mice and n =13 neurons/6 mice for WT and KO neurons, respectively) were modified between genotypes, suggesting a normal postsynaptic function in KO mice ( Fig. 1d ). The slower decay kinetics of evoked responses with respect to the miniature currents in WT neurons has been previously attributed to higher level of asynchronous vesicle release [28] . Thus, these data suggest that the absence of Syn II favours synchronous release at dentate gyrus inhibitory synapses. Short-term plasticity in Syn II KO neurons The data reported in Fig. 1 suggest that SVs in inhibitory nerve terminals of KO mice are more prone to undergo exocytosis in response to a sudden increase in Ca 2+ following the action potential. We tested this possibility by using a paired-pulse stimulation protocol, which is tightly affected by changes in the intraterminal Ca 2+ concentration [29] , [30] . The paired-pulse depression (PPD) induced at short inter-stimulus intervals (ISIs) was similar between genotypes at short ISIs, but it significantly increased in KOs when ISIs were increased to 2 or 3 s ( Fig. 2a ). PPD at short ISIs (PPD fast ) is highly dependent on Ca 2+ , while at longer ISIs (PPD slow ) the Ca 2+ -dependence is progressively lost [29] . Thus, the more intense PPD slow observed in the KO slices, could result from a larger depletio of the SV pool induced by the first stimulation, whose amplitude was larger in KO than in WT neurons. To evaluate this possibility, we compared the normalized amplitudes of the first and second responses at 2-s ISI [29] , [31] ( Fig. 2c ) and further evaluated synaptic depression in response to different trains of stimuli ( Figs 2e and 3a ). The lack of correlation between the two parameters suggests that the depression of the second eIPSC is independent of the amount of SVs released by the first stimulus ( Fig. 2c ). Next, we investigated whether PPD had either a presynaptic or postsynaptic origin. The variation in the peak current amplitude during the first and second IPSCs was evaluated for inter-pulse intervals of 2 and 3 s (12 pairs for WT and 16 pairs for KO using an analysis developed by Malinow and Tsien [31] , [32] (see Methods). 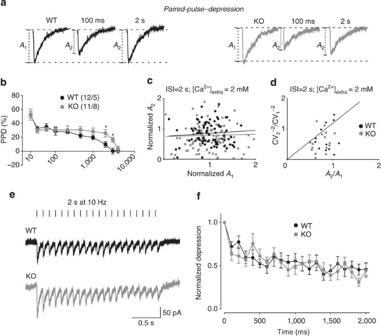Figure 2: Syn II deletion does not induce major changes in short-term plasticity at inhibitory synapses. (a) Representative dual eIPSCs traces recorded from dentate gyrus WT (black) and KO (grey) neurons in response to paired stimulation of the medial perforant path at the indicated ISIs. (b) The mean per cent (±s.e.m.) PPD observed in WT (black symbols;n=8–12) and KO (grey symbols;n=6–13) neurons is plotted as a function of the ISI. (c) Plot of the amplitude of the response to the second pulse (A2) versus the amplitude of the response to the first pulse (A1) (10 responses/neuron fromn=13 KO and 12 WT neurons,) at 2-s ISI in 2 mM Ca2+. Both amplitudes are normalized to the meanA1in the recorded ensemble. Linear regression analysis of the data points (black and grey lines for WT and KO, respectively) shows no significant correlation betweenA1andA2. (d) The inverse of the square coefficient of variation (CV−2) of the second IPSC (A2) normalized by the CV1of the first IPSC (A1) was plotted against the PPR (A2/A1) (n=12 andn=16 pairs of WT and KO neurons stimulated at 2 s ISI, respectively). Note that most of the data points of both WT and KO neurons fall below the unitary line, indicating a presynaptic mechanism of short-term depression. (e) Representative traces from WT (black) and KO (grey) in response to stimulation of the medial perforant path for 2 s at 10 Hz. (f) Plot of normalized peak amplitude (±s.e.m.) versus time showing the multiple-pulse depression at 10 Hz in WT (black) and KO (grey) neurons. Figure 2d shows a summary plot of the inverse of the square of the CV (CV −2 ) versus the mean amplitude of the second response, both normalized to the values of the first IPSC for both WT and KO neurons. Most of the experimental points fell under the identity line, indicating a presynaptic origin of the increased PPD slow observed in KO slices. Several studies report that the lack of Syns causes higher depression in response to various stimulation frequencies in both excitatory and inhibitory synapses [17] , [25] . In contrast, we observed that Syn II deletion had no effects on synaptic depression induced by stimulation at either 10 or 40 Hz in both inhibitory ( Figs 2e , f and ) and excitatory ( Supplementary Fig. S3a–c ) synapses. Figure 2: Syn II deletion does not induce major changes in short-term plasticity at inhibitory synapses. ( a ) Representative dual eIPSCs traces recorded from dentate gyrus WT (black) and KO (grey) neurons in response to paired stimulation of the medial perforant path at the indicated ISIs. ( b ) The mean per cent (±s.e.m.) PPD observed in WT (black symbols; n =8–12) and KO (grey symbols; n =6–13) neurons is plotted as a function of the ISI. ( c ) Plot of the amplitude of the response to the second pulse ( A 2 ) versus the amplitude of the response to the first pulse ( A 1 ) (10 responses/neuron from n =13 KO and 12 WT neurons,) at 2-s ISI in 2 mM Ca 2+ . Both amplitudes are normalized to the mean A 1 in the recorded ensemble. Linear regression analysis of the data points (black and grey lines for WT and KO, respectively) shows no significant correlation between A 1 and A 2 . ( d ) The inverse of the square coefficient of variation (CV −2 ) of the second IPSC ( A 2 ) normalized by the CV 1 of the first IPSC ( A 1 ) was plotted against the PPR ( A 2 / A 1 ) ( n =12 and n =16 pairs of WT and KO neurons stimulated at 2 s ISI, respectively). Note that most of the data points of both WT and KO neurons fall below the unitary line, indicating a presynaptic mechanism of short-term depression. ( e ) Representative traces from WT (black) and KO (grey) in response to stimulation of the medial perforant path for 2 s at 10 Hz. ( f ) Plot of normalized peak amplitude (±s.e.m.) versus time showing the multiple-pulse depression at 10 Hz in WT (black) and KO (grey) neurons. 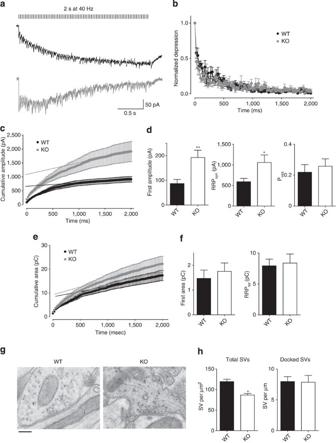Figure 3: Syn II deletion increases the RRP size of synchronously released GABA vesicles. (a) Representative responses from WT (black) and KO (grey) neurons induced by stimulation of the medial perforant path for 2 s at 40 Hz. Stimulation artifacts were removed for clarity. (b) Plot of the normalized amplitude (means±s.e.m.) versus time showing the multiple-pulse depression during the 40-Hz train in WT (black) and KO (grey) neurons. (c) Cumulative amplitude profile of a 2-s train at 40 Hz. Data points from the last second of the response were fitted by linear regression and the line was extrapolated to time 0 to estimate the RRPsyn. (d) Mean values (±s.e.m.) of the amplitude of the first eIPSC in the train, RRPsynandPvesfor WT (black bars) and KO (open bars) neurons. (e) Cumulative area profile of a 2-s train at 40 Hz. Data points from the last second of the response were fitted by linear regression and the line was extrapolated to time 0 to estimate the RRPtot. (f) Mean values (±s.e.m.) of the first eIPSC area in the train and RRPtotfor WT (black bars) and KO (open bars) neurons. For electrophysiology experiments: **P<0.01, two-tailed unpaired Student’st-test and *P<0.05, Welch’st-test.n=16 andn=14 neurons from WT (5 mice) and KO (8 mice), respectively. (g) Micrographs of GABA-immunopositive synaptic terminals (stained by 10 nm gold particles) making contact with granule cell dendrites in the molecular layer of the dentate gyrus of WT and KO slices. Scale bar, 200 nm. (h) Mean values (±s.e.m.) of the density of total SVs and the number of docked SVs in presynaptic terminals of WT (black bars) and KO (open bars) neurons. For EM experiments: *P<0.05, unpaired Student’st-test;n=100/39 synapses from 4 WT mice and 69/72 synapses from 4 KO mice. Full size image Figure 3: Syn II deletion increases the RRP size of synchronously released GABA vesicles. ( a ) Representative responses from WT (black) and KO (grey) neurons induced by stimulation of the medial perforant path for 2 s at 40 Hz. Stimulation artifacts were removed for clarity. ( b ) Plot of the normalized amplitude (means±s.e.m.) versus time showing the multiple-pulse depression during the 40-Hz train in WT (black) and KO (grey) neurons. ( c ) Cumulative amplitude profile of a 2-s train at 40 Hz. Data points from the last second of the response were fitted by linear regression and the line was extrapolated to time 0 to estimate the RRP syn . ( d ) Mean values (±s.e.m.) of the amplitude of the first eIPSC in the train, RRP syn and P ves for WT (black bars) and KO (open bars) neurons. ( e ) Cumulative area profile of a 2-s train at 40 Hz. Data points from the last second of the response were fitted by linear regression and the line was extrapolated to time 0 to estimate the RRP tot . ( f ) Mean values (±s.e.m.) of the first eIPSC area in the train and RRP tot for WT (black bars) and KO (open bars) neurons. For electrophysiology experiments: ** P <0.01, two-tailed unpaired Student’s t -test and * P <0.05, Welch’s t -test. n =16 and n =14 neurons from WT (5 mice) and KO (8 mice), respectively. ( g ) Micrographs of GABA-immunopositive synaptic terminals (stained by 10 nm gold particles) making contact with granule cell dendrites in the molecular layer of the dentate gyrus of WT and KO slices. Scale bar, 200 nm. ( h ) Mean values (±s.e.m.) of the density of total SVs and the number of docked SVs in presynaptic terminals of WT (black bars) and KO (open bars) neurons. For EM experiments: * P <0.05, unpaired Student’s t -test; n =100/39 synapses from 4 WT mice and 69/72 synapses from 4 KO mice. Full size image Syn II deletion enhances the synchronous RRP Based on the previous observations, we then investigated the properties of the synchronous and asynchronous GABA release by using high-frequency stimulation. By analysing the cumulative amplitude profile during a high-frequency train (2 s at 40 Hz; Fig. 3c ), we observed a larger amplitude of the first response in the train in KO neurons (86.86±16.86, n =16 neurons/5 mice and 192.3±29.56 pA; n =14 neurons/8 mice for WT and KO neurons, respectively, P =0.003; Fig. 3d ). Such increase of the synchronous response is due to an increase in the readily releasable pool size (RRP syn ) (591.8±79.5 versus 1,058.0±181.9 pA, for WT and KO neurons respectively, P =0.02) and not to a change in the vesicular release probability ( P ves ) (0.21±0.04 versus 0.25±0.04, for WT and KO neurons respectively, P =0.56; Fig. 3d ). We further studied the quantal parameters of inhibitory synaptic transmission using the multiple fluctuation probability analysis [17] . This method ( Supplementary Methods ), that provides direct information on the average quantal release probability (Pr av ), number of independent release sites ( N min ) and average postsynaptic quantal size ( Q av ), fully confirmed the data obtained by the cumulative amplitude analysis indicating that an increase in N min is responsible for the increased eIPSC amplitude ( Supplementary Fig. S4 ). However, the RRP size determined with these methods is an underestimation of the total RRP, as it represents only the synchronously released part of SVs [33] . The cumulative area method gives a better estimation of the total RRP [33] , as it includes also the asynchronous component of the response ( Fig. 3e ). Not only the area of the first response of the train did not change between genotypes (1.47±0.33 and 1.75±0.33 pC, for WT and KO neurons, respectively, P =0.55) ( Figs 3f and 1b ), but also the RRP tot , measured with the cumulative area method, resulted similar between genotypes (7.93±1.07 and 8.37±1.46 pC, for WT and KO neurons, respectively, P =0.80; Fig. 3f ). We next used electron microscopy ( Supplementary Methods ) to morphologically evaluate the number and spatial distribution of SVs within the inhibitory GABA-immunopositive terminals in the molecular layer of the dentate gyrus of KO and WT slices ( Fig. 4g ). The total density of SVs was significantly decreased in KO synapses (120.8±9.1, n =100 terminals/4 mice and 88.2±3.9 SVs per μm 2 , n =69 terminals/4 mice, for WT and KO, respectively, P =0.016; Fig. 3g ). However, the number of docked SVs, putatively corresponding to the functional RRP [34] , did not differ between genotypes (7.97±0.80, n =39 terminals/4 mice, and 7.85±1.11 SVs per μm, n =72 terminals/4 mice, for WT and KO, respectively, P =0.93) ( Fig. 3g ). Together, these results strengthen the indication that the synchronous and asynchronous release appear to compete for a common pool of release-ready SVs [35] and that the ratio between the two modalities of release is modified in the absence of Syn II. 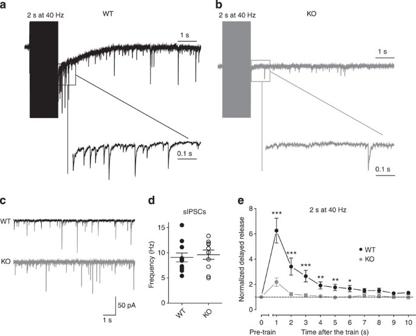Figure 4: Syn II deletion dramatically reduces the delayed asynchronous GABA release. (a,b) Representative traces of the inhibitory delayed asynchronous response in WT (a; black) and KO (b; grey) dentate gyrus granule cells after stimulation of the medial perforant path. Inset traces represent the first second after the end of the stimulation. (c) Representative traces of sIPSCs recorded in dentate gyrus granule neurons from WT (black) and KO (grey) mice. (d) Frequency (means±s.e.m.) of sIPSC measured at −80 mV in the presence of 50 μM D-APV, 10 μM CNQX, 5 μM CGP 55845 (n=11 andn=10 neurons from 5 WT mice and 9 KO mice, respectively). Each dot represents a single experiment. (e) Plot of the mean (±s.e.m.) charge of the delayed GABA release as a function of time after the end of the stimulation train. Data (black and grey symbols/lines for WT and KO, respectively) were normalized to the pre-train spontaneous release. *P<0.05, **P<0.01 and ***P<0.001, Welch’st-test.n=26 andn=24 neurons from WT (10 mice) and KO (12 mice), respectively. Figure 4: Syn II deletion dramatically reduces the delayed asynchronous GABA release. ( a , b ) Representative traces of the inhibitory delayed asynchronous response in WT ( a ; black) and KO ( b ; grey) dentate gyrus granule cells after stimulation of the medial perforant path. Inset traces represent the first second after the end of the stimulation. ( c ) Representative traces of sIPSCs recorded in dentate gyrus granule neurons from WT (black) and KO (grey) mice. ( d ) Frequency (means±s.e.m.) of sIPSC measured at −80 mV in the presence of 50 μM D-APV, 10 μM CNQX, 5 μM CGP 55845 ( n =11 and n =10 neurons from 5 WT mice and 9 KO mice, respectively). Each dot represents a single experiment. ( e ) Plot of the mean (±s.e.m.) charge of the delayed GABA release as a function of time after the end of the stimulation train. Data (black and grey symbols/lines for WT and KO, respectively) were normalized to the pre-train spontaneous release. * P <0.05, ** P <0.01 and *** P <0.001, Welch’s t -test. n =26 and n =24 neurons from WT (10 mice) and KO (12 mice), respectively. Full size image Delayed asynchronous release is reduced in Syn II KO mice High-frequency stimulation trains lead to delayed asynchronous release that persists for tens/hundreds of milliseconds to seconds in excitatory and inhibitory synapses [4] , [5] , [7] , [36] . Thus, we measured the delayed asynchronous release in response to trains of 40 Hz ( Fig. 4a ). The extent of spontaneous network activity preceding the application of the train may influence the amount of asynchronous release induced by the train. To eliminate this possibility, we measured the frequency of spontaneous IPSCs (sIPSCs) before the train stimulus, and observed similar values in the two genotypes (9.07±0.87, n =11 neurons/5 mice and 9.61±0.93, n =10 neurons/9 mice for WT and KO neurons, respectively, P =0.67; Fig. 4c ). WT synapses showed enhanced asynchronous release after the train that slowly returned to baseline within 10 s, while in KO synapses the asynchronous release was tenfold lower and returned to baseline value within 2 s after the train ( Fig. 4e ). The delayed asynchronous release at excitatory synapses was not altered in KO neurons ( Supplementary Fig. S3d ), indicating the specificity of this phenotype for inhibitory synapses. The virtual absence of delayed asynchronous release of GABA may participate in the development of the strong epileptic phenotype of adult Syn II KO mice. Thus, we repeated the experiments in the dentate gyrus of adult symptomatic mice and found a closely similar depression of the delayed asynchronous release of GABA ( Supplementary Fig. S5 ). It was of interest to check whether Syn I, the most abundant Syn isoform, had any effect in the modulation of asynchronous release. Interestingly, we observed that Syn I deletion increased the asynchronous release in inhibitory synapses of primary hippocampal neurons, conforming with a non-redundant function of Syn I on release dynamics that is opposite to that of Syn II ( Supplementary Fig. S6 ). Moreover, the increase in the asynchronous response of Syn I KO inhibitory neurons was associated with decreased eIPSC amplitude and RRP size [17] , which are opposite respect to the changes observed in Syn II KO neurons ( Figs 1 and 3 ). Syn II modulates release in a Ca 2+ -dependent manner Both synchronous and asynchronous release are Ca 2+ -dependent, but they are likely to be mediated by two distinct Ca 2+ sensors with different Ca 2+ affinities: a low-affinity sensor that sustains fast synchronous release and a high-affinity sensor that is involved in the slow asynchronous release [7] , [8] . We attempted to experimentally desynchronize the inhibitory synaptic transmission by replacing extracellular Ca 2+ with Sr 2+ , as the distinct Ca 2+ sensors have the same affinity for Sr 2+ ( [4] , [37] , [38] , [39] ). In the single-pulse protocol, Sr 2+ (2 mM) induced a reduction in the peak amplitude of the synchronous current in both WT (106.31±26.36 versus 56.42±12.06 pA, P =0.018, n =5 neurons/3 mice) and KO neurons (245.62±37.16 versus 87.99±20.49 pA, P =0.005, n =4 neurons/3 mice) ( Fig. 5a ). However, the per cent reduction in the peak amplitude induced by Sr 2+ was higher in KO than in WT neurons (45.48±6.050% and 64.99±4.997%, for WT and KO, respectively, P =0.047; Fig. 5c ). Also, the fast component ( τ fast ) of the response in Sr 2+ had similar values as in Ca 2+ and was unchanged between genotypes (9.94±5.35 and 9.85±3.84 ms for WT and KO neurons, respectively, P =0.99), while the slow component ( τ slow ) of the decay was significantly slower in Sr 2+ , yet still unchanged between WT and KO neurons (84.27±37.78 and 63.11±32.16 ms, for WT and KO neurons, respectively, P =0.69; Fig. 5d ). Changing the extracellular solution from Ca 2+ to Sr 2+ severely desynchronized the sIPSCs in both WT and KO neurons, but when high-frequency stimulation trains were applied in the presence of Sr 2+ , a significant increase in the delayed asynchronous release was observed only in KO neurons ( Fig. 5e ). 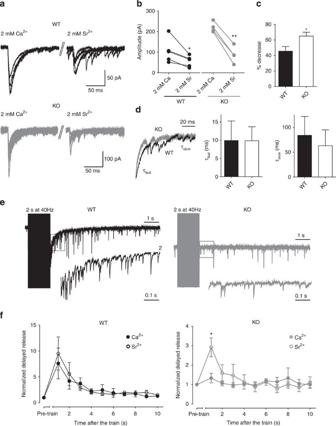Figure 5: Ca2+-dependency of delayed asynchronous GABA release in Syn II KO neurons. (a) Representative traces of eIPSCs from the same WT (black) and KO (grey) dentate gyrus granule neurons in 2 mM Ca2+and after replacement of Ca2+with 2 mM Sr2+. (b) Plot of the peak amplitude of eIPSCs before and after the switch to 2 mM Sr2+for WT (black) and KO (grey) neurons. (c) Mean values (±s.e.m.) of the per cent depression in the peak eIPSC amplitude for WT and KO neurons (closed and open bars, respectively) after replacement of Ca2+with Sr2+. (d) Representative traces of the eIPSC decay. The trace recorded in WT neurons (black) was normalized to the peak amplitude of eIPSC in KO neurons (grey trace) in 2 mM Sr2+. A two-exponential model was used to fit the fast and the slow components of the decay (τfastandτslow). *P<0.05 and **P<0.01, two-tailed paired (b) and unpaired (c) Student’st-test.n=5 andn=4 neurons from WT (3 mice) and KO (3 mice), respectively. (e) Representative traces of the delayed asynchronous inhibitory response in 2 mM Sr2+recorded in WT (black) and KO (grey) dentate gyrus granule neurons after stimulation of the medial perforant path. Inset traces represent the first second after the end of the stimulation. (f) Plots of the mean (±s.e.m.) charge of the delayed asynchronous release as a function of time after the end of the stimulation train in WT and KO neurons. Data recorded in the presence of either 2 mM Ca2+(closed symbols) or 2 mM Sr2+(open symbols) were normalized to the respective pre-train spontaneous release. *P<0.05, two-tailed paired Student’st-testn=11 andn=4 neurons from WT (3 mice) and KO (3 mice), respectively. Figure 5: Ca 2+ -dependency of delayed asynchronous GABA release in Syn II KO neurons. ( a ) Representative traces of eIPSCs from the same WT (black) and KO (grey) dentate gyrus granule neurons in 2 mM Ca 2+ and after replacement of Ca 2+ with 2 mM Sr 2+ . ( b ) Plot of the peak amplitude of eIPSCs before and after the switch to 2 mM Sr 2+ for WT (black) and KO (grey) neurons. ( c ) Mean values (±s.e.m.) of the per cent depression in the peak eIPSC amplitude for WT and KO neurons (closed and open bars, respectively) after replacement of Ca 2+ with Sr 2+ . ( d ) Representative traces of the eIPSC decay. The trace recorded in WT neurons (black) was normalized to the peak amplitude of eIPSC in KO neurons (grey trace) in 2 mM Sr 2+ . A two-exponential model was used to fit the fast and the slow components of the decay ( τ fast and τ slow ). * P <0.05 and ** P <0.01, two-tailed paired ( b ) and unpaired ( c ) Student’s t -test. n =5 and n =4 neurons from WT (3 mice) and KO (3 mice), respectively. ( e ) Representative traces of the delayed asynchronous inhibitory response in 2 mM Sr 2+ recorded in WT (black) and KO (grey) dentate gyrus granule neurons after stimulation of the medial perforant path. Inset traces represent the first second after the end of the stimulation. ( f ) Plots of the mean (±s.e.m.) charge of the delayed asynchronous release as a function of time after the end of the stimulation train in WT and KO neurons. Data recorded in the presence of either 2 mM Ca 2+ (closed symbols) or 2 mM Sr 2+ (open symbols) were normalized to the respective pre-train spontaneous release. * P <0.05, two-tailed paired Student’s t -test n =11 and n =4 neurons from WT (3 mice) and KO (3 mice), respectively. Full size image To further confirm the Ca 2+ dependency of the Syn II, we analysed the amplitude of the evoked response and the delayed asynchronous release in different extracellular Ca 2+ concentrations ( Fig. 6 ). At low Ca 2+ concentrations, (0.5 and 1 mM) both the eIPSC amplitude and the delayed asynchronous release (measured here only for the first second after the train for simplicity) were not changed between WT and KO mice ( Fig. 6a ). However, a clearly distinct behaviour of the analysed parameters was observed at higher Ca 2+ (4 and 6 mM). While the amplitude of eIPSC increased linearly with the Ca 2+ concentration in the KO mice, remaining significantly higher than the WT ( Fig. 6c ), the delayed asynchronous response of KO neurons remained at basal levels and was completely insensitive to the increasing Ca 2+ concentration ( Fig. 6d ). On the contrary, short-term plasticity in WT and KO inhibitory responses was not affected by the different Ca 2+ levels ( Supplementary Fig. S7 ). Taken together, these data further demonstrate that the absence of Syn II from inhibitory synapses abolishes the delayed asynchronous release in favour of evoked synchronous release. 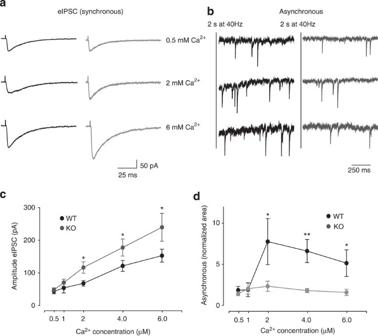Figure 6: Syn II deletion modulates the synchronous/asynchronous release in a Ca2+-dependent manner. (a) Representative traces of eIPSCs from WT (black) and KO (grey) dentate gyrus neurons at low (0.5 mM), normal (2 mM) and high (6 mM) extracellular Ca2+concentrations. (b) Representative traces of the first second after a 2-s train at 40 Hz from WT (black) and KO (grey) neurons at different Ca2+concentrations. (c,d) eIPSCs peak amplitude (c) and normalized area of the first second after the train (d) in WT and KO slices as a function of the increasing extracellular Ca2+concentration. *P<0.05, **P<0.01, Welch’st-test.n=10 neurons/6 mice for WT andn=9 neurons/5 mice for KO. Figure 6: Syn II deletion modulates the synchronous/asynchronous release in a Ca 2+ -dependent manner. ( a ) Representative traces of eIPSCs from WT (black) and KO (grey) dentate gyrus neurons at low (0.5 mM), normal (2 mM) and high (6 mM) extracellular Ca 2+ concentrations. ( b ) Representative traces of the first second after a 2-s train at 40 Hz from WT (black) and KO (grey) neurons at different Ca 2+ concentrations. ( c , d ) eIPSCs peak amplitude ( c ) and normalized area of the first second after the train ( d ) in WT and KO slices as a function of the increasing extracellular Ca 2+ concentration. * P <0.05, ** P <0.01, Welch’s t -test. n =10 neurons/6 mice for WT and n =9 neurons/5 mice for KO. Full size image Syn II interacts with Ca2 + channels to modulate GABA release While Syn I displays a Ca 2+ -binding site involving a glutamate residue (E373), Syn II does not share this key acidic residue indispensable for Ca 2+ coordination and has a basic residue instead (K374) [40] . On this basis, Syn II is predicted not to bind Ca 2+ and, accordingly, ATP binding to Syn II is not Ca 2+ -dependent [40] . Thus, Syn II cannot theoretically control asynchronous release by direct binding of Ca 2+ . However, recent data by proteomics [41] reported that Syn I and Syn II may interact with Ca 2+ channels. To confirm this possibility, we performed functional experiments with blockers of distinct subtypes of presynaptic Ca 2+ currents. Addition of ω-Agatoxin-IVA, a blocker of P/Q-type Ca 2+ currents, reduced the peak amplitude of the GABA synchronous response by 50% in both phenotypes (49.9±13.04% and 50.0±12.64%, n =6 neurons/4 mice and n =5 neurons/4 mice for WT and KO, respectively, P =0.99; Fig. 7a ). Similarly, addition of ω-Conotoxin-GVIA, a blocker of N-type Ca 2+ currents, caused a similar ~50% reduction in the amplitude of the GABA synchronous current in both WT and KO neurons (51±10.33% and 56.75±7.98%, n =5 neurons/5 mice and n =6 neurons/3 mice for WT and KO, respectively, P =0.670; Fig. 7a ). Importantly, neither ω-Agatoxin-IVA nor ω-Conotoxin-GVIA had any effect on the delayed asynchronous release in Syn II KO neurons, but reduced it significantly in WT slices ( Fig. 7c–e ). To further support these functional data, we performed co-immunoprecipitation experiments on cortical neuron lysates, using anti-Syn I and anti-Syn II antibodies. While no interaction was present between Syn II and Cav2.2 (N-type)/ Cav2.3 (R-type) channels, a specific interaction was detected between Syn II and Cav2.1 (P/Q-type; Fig. 7f ). Interestingly, the interaction appeared to be specific for Syn II, as virtually no interaction between Syn I and all tested Ca 2+ channels was detected ( Supplementary Fig. S8 ). Taken together, these data suggest that Syn II controls the amount of asynchronous release at inhibitory synapses through an interaction with a specific subtype of Ca 2+ channels. 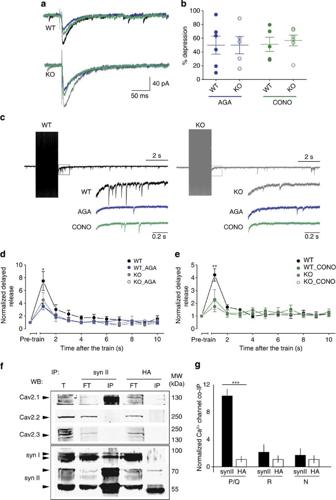Figure 7: Syn II modulates GABA asynchronous release by interacting with presynaptic Ca2+channels. (a) Representative traces of eIPSCs from WT and KO dentate gyrus granule neurons before (black and grey for WT and KO, respectively) and after blockade of P/Q-type Ca2+current with 0.5 μM ω-Agatoxin-IVA (blue) or of N-type Ca2+current with 1 μM ω-Conotoxin-GVIA (green). (b) Aligned dot plot of the per cent reduction in peak amplitude of eIPSCs in WT (closed circles) and KO (open circles) neurons after the addition of either ω-Agatoxin-IVA (AGA; 0.5 μM) or ω-Conotoxin-GVIA (CONO; 1 μM). (c) Representative traces of the delayed asynchronous inhibitory response in WT and KO neurons (black and grey, respectively) and its modulation by Ca2+-channel blockers. Inset traces represent the first second after the end of the stimulation under control conditions and after the addition of ω-Agatoxin-IVA (0.5 μM; blue) or ω-Conotoxin-GVIA (1 μM; green). (d) Plots of the mean (±s.e.m.) charge of the delayed asynchronous release as a function of time after the end of the stimulation train in WT and KO neurons. Data recorded under control conditions (black/grey circles) or in the presence of ω-Agatoxin-IVA (0.5 μM; closed/open blue circles) were normalized to the respective pre-train spontaneous release. *P<0.05, two-tailed paired Student’st-test.n=5 neurons from both WT (4 mice) and KO (4 mice), respectively. (e) Same as ford, but in the presence of ω-Conotoxin-GVIA (1 μM; closed/open green circles) **P<0.01, two-tailed paired Student’st-test.n=5 andn=6 neurons from WT (4 mice) and KO (3 mice), respectively. (f,g) Cortical neuron lysates were immunoprecipitated with anti-SynII antibodies or anti-HA antibodies, as indicated (immunoprecipitation (IP)). After electrophoretic separation of the immunocomplexes, membranes were probed with antibodies specific for anti-Cav2.1 (P/Q-type), anti-Cav2.2 (N-type) and anti-Cav2.3 (R-type) Ca2+channel subunits, as indicated (western blotting (WB)). A representative immunoblot is shown (f), together with the quantification of the immunoreactive signal in the immunoprecipitated samples (g), normalized to the binding to the HA control (means±s.e.m.;n=3 independent experiments). T, 100 μg of total lysate; FT, 100 μg of flow-through after immunoprecipitation. Figure 7: Syn II modulates GABA asynchronous release by interacting with presynaptic Ca 2+ channels. ( a ) Representative traces of eIPSCs from WT and KO dentate gyrus granule neurons before (black and grey for WT and KO, respectively) and after blockade of P/Q-type Ca 2+ current with 0.5 μM ω-Agatoxin-IVA (blue) or of N-type Ca 2+ current with 1 μM ω-Conotoxin-GVIA (green). ( b ) Aligned dot plot of the per cent reduction in peak amplitude of eIPSCs in WT (closed circles) and KO (open circles) neurons after the addition of either ω-Agatoxin-IVA (AGA; 0.5 μM) or ω-Conotoxin-GVIA (CONO; 1 μM). ( c ) Representative traces of the delayed asynchronous inhibitory response in WT and KO neurons (black and grey, respectively) and its modulation by Ca 2+ -channel blockers. Inset traces represent the first second after the end of the stimulation under control conditions and after the addition of ω-Agatoxin-IVA (0.5 μM; blue) or ω-Conotoxin-GVIA (1 μM; green). ( d ) Plots of the mean (±s.e.m.) charge of the delayed asynchronous release as a function of time after the end of the stimulation train in WT and KO neurons. Data recorded under control conditions (black/grey circles) or in the presence of ω-Agatoxin-IVA (0.5 μM; closed/open blue circles) were normalized to the respective pre-train spontaneous release. * P <0.05, two-tailed paired Student’s t- test. n =5 neurons from both WT (4 mice) and KO (4 mice), respectively. ( e ) Same as for d , but in the presence of ω-Conotoxin-GVIA (1 μM; closed/open green circles) ** P <0.01, two-tailed paired Student’s t -test. n =5 and n =6 neurons from WT (4 mice) and KO (3 mice), respectively. ( f , g ) Cortical neuron lysates were immunoprecipitated with anti-SynII antibodies or anti-HA antibodies, as indicated (immunoprecipitation (IP)). After electrophoretic separation of the immunocomplexes, membranes were probed with antibodies specific for anti-Cav2.1 (P/Q-type), anti-Cav2.2 (N-type) and anti-Cav2.3 (R-type) Ca 2+ channel subunits, as indicated (western blotting (WB)). A representative immunoblot is shown ( f ), together with the quantification of the immunoreactive signal in the immunoprecipitated samples ( g ), normalized to the binding to the HA control (means±s.e.m. ; n =3 independent experiments). T, 100 μg of total lysate; FT, 100 μg of flow-through after immunoprecipitation. Full size image We examined the dynamics of basal neurotransmitter release and short-term plasticity in mouse hippocampal inhibitory synapses lacking Syn II. For the first time, we report that Syn II has a specific post-docking role in inhibitory synapses, influencing basal GABA release and leading to subtle changes in short-term plasticity ( Figs 1 , 2 and 3 ). More importantly, Syn II appears to modify the dynamics of GABA release by promoting asynchronous SV release at the expense of synchronous release ( Fig. 4 ). Finally, we demonstrate that Syn II interacts with presynaptic Ca 2+ channels to promote GABA asynchronous release ( Figs 5 , 6 and 7 ). Inhibitory synapses lacking Syn I, Syn III or all three Syn isoforms show a decrease in the amplitude of the IPSCs evoked by single action potentials [16] , [17] , [42] , [43] . We have found that the deletion of Syn II increases the peak amplitude of evoked responses and reduces the frequency of the mIPSCs at hippocampal inhibitory synapses. Opposite to the findings from Syn I KO mice in which synaptic depression at inhibitory synapses was enhanced [17] , the Syn II deletion lead to no changes in synaptic depression and minute changes in PPD. These data suggest that the various Syn isoforms are endowed with distinct post-docking functions at inhibitory synapses. The increased inhibitory response to single stimulation in Syn II KO neurons appears to be induced by acceleration of the dynamics of GABA release. Deletion of SYN2 strongly enhanced synchronous SV release, while the delayed asynchronous release was virtually abolished. These results imply that the function of Syn II is to desynchronize SV release, opposite to Syn I that was hypothesized to facilitate release synchronization [44] , [45] . Indeed, we found that deletion of Syn I increased the asynchronous release in inhibitory synapses, an effect opposite to that of Syn II deletion. Thus, the possibility exists that Syns I and II have non-redundant functions and constitute a push–pull mechanism regulating the ratio between synchronous and asynchronous release in the synapses in which they are co-expressed. An important question is how Syn II changes the ratio between synchronous and asynchronous neurotransmitter release. As both Syn I and Syn II do not apparently affect the pool of docked SVs, we suggest that they might directly affect downstream exocytotic events and regulate the dynamics of release. The synchronous release has been so far connected with members of the synaptotagmin family of Ca 2+ sensors [9] , [10] , [11] . Synaptotagmin-1 or synaptotagmin-2 deletions lead to a complete loss of synchronous release at both excitatory and inhibitory synapses [9] , [10] , [11] , while asynchronous release is preserved and even enhanced at high stimulation frequencies [10] . The knockdown of synaptotagmin-7 at the zebrafish neuromuscular junction reduces asynchronous release [46] , however it has no effect on synchronous/asynchronous release in central synapses [47] . We detected no interaction of either Syn I or Syn II with the various synaptotagmin isoforms (−1, −2 and −7) in coimmunoprecipitation experiments (data not shown), suggesting that the accelerated neurotransmitter release in Syn KO II slices is independent of a possible impairment of the synaptotagmin normal function. On the other hand, the mechanisms behind asynchronous release are still far from being understood, with recent work proposing several hypotheses. One proposed mechanism involves a slow presynaptic Ca 2+ sensor, Doc2, that binds Ca 2+ with slower kinetics and its knockdown in hippocampal cultures results in reduced asynchronous release [48] . Another recent paper reports that the SNARE protein VAMP2 drives synchronous release, while its isoform VAMP4 boosts asynchronous release [14] . Moreover, it was recently shown that both voltage-gated presynaptic Cav-2.1 and Cav-2.2 channels, that conduct P/Q-type and N-type Ca 2+ currents respectively, are characterized by a prolonged Ca 2+ current that promotes asynchronous release [49] . The sensitivity of both evoked synchronous and delayed asynchronous release to Sr 2+ versus Ca 2+ and to various concentrations of extracellular Ca 2+ in Syn II KO slices supports the idea that the postdocking functions of Syn II are Ca 2+ dependent. One possible explanation for this Ca 2+ -dependency is that Syns modulate neurotransmitter release by coupling SVs with presynaptic Ca 2+ channels. Indeed, several studies demonstrated that Ca 2+ channels are tightly coupled with SVs in the nanodomain range [50] and, in addition, a potential interaction between Syn I and Syn II with distinct Ca 2+ channel subunits was recently reported by means of proteomics [41] . In our experiments, addition of blockers of either P/Q- or N-type of Ca 2+ currents reduced the synchronously evoked and delayed asynchronous current in WT slices, but the delayed asynchronous release was not affected by both Ca 2+ -channel blockers in Syn II KO slices. Our patch-clamp experiments were performed at non-specific hippocampal inhibitory synapses, where at least a subset includes output synapses from interneurons expressing P/Q or N-type Ca 2+ channels, as Ca 2+ channels are interneuron specific [2] , [50] . Interestingly, we found for the first time that, Syn II specifically interacts with Cav-2.1 type Ca 2+ channels, but not with Cav-2.2 or Cav-2.3 types, while Syn I does not co-immunoprecipitate with any of the main presynaptic Ca 2+ -channel subunits, indicating a physiologically important and non-redundant function of Syn II with respect to Syn I. We cannot exclude that the interaction between Syn II and Cav-2.1 type Ca 2+ -channels is indirect and mediated by modulatory proteins of the active zone, such as via the Rab3-RIM-Ca 2+ -channel pathway. This hypothesis is supported by the fact that Syns interact with Rab3 [51] , [52] and may thereby interfere with RIM binding to N and P/Q-type Ca 2+ channels at the active zone [53] , decreasing the efficiency, speed and synchrony of release. As Syn II appears to bind more tightly to SVs than Syn I (F. Benfenati, unpublished observations), it is possible that Syn II remains to a large extent attached to SVs during the post-docking steps of release, possibly acting as a brake for the synchronous release of SVs docked in the vicinity of a specific Ca 2+ channel. The genetic deletion of Syn II may decrease the physical distance between Ca 2+ channels and SVs at GABAergic synapses, thus speeding up neurotransmitter release with respect to the incoming action potential. Under these conditions, if a train of action potentials invades the presynaptic site, then the SVs available for release are more rapidly exhausted, thus explaining the lack of delayed asynchronous release in the Syn II KO neurons. Although Syn II specifically interacts only with P/Q-type Ca 2+ channels, its deletion occluded the effects of both P/Q- and N-type Ca 2+ channel blockers. This suggests that the Syn II effect on the asynchronous release is downstream of the asynchronous Ca 2+ current, and that both types of channels contribute to the bulk intraterminal Ca 2+ that drives asynchronous release. Strikingly, the effect of Syn II deletion was restricted to inhibitory neurons, and no effects on release dynamics or short-term plasticity were observed in excitatory synapses. We demonstrated that, in inhibitory neurons, the effects of Syn II deletion on release dynamics occur only at physiological Ca 2+ concentrations, while decreasing extracellular Ca 2+ to decrease Pr virtually abolishes this phenotype ( Fig. 6 ). It is therefore possible that the effects of Syn II on release dynamics require high Pr values and therefore emerge under physiological Ca 2+ conditions in inhibitory synapses, but not in excitatory synapses that are characterized by significantly lower Pr values [54] , [55] . This desynchronizing effect of Syn II on inhibitory synapses may have pathologic consequences, as Syn II KO mice are epileptic, with seizures starting after 2–3 months of life [25] , [56] . Changes in GABA asynchronous release between specific neurons from human epileptic and non-epileptic tissue have been recently reported [57] . After trains of APs or in some cases just one AP, long-lasting IPSCs generated by asynchronous GABA release occurring with significant delays can increase the effectiveness of inhibition [58] , [59] . Asynchronous GABA release apparently allows an inhibitory compensatory tuning proportional to the extent of presynaptic activity, and is markedly increased when synapses are stimulated with behaviourally relevant high-frequency patterns [5] , [36] . Interestingly, we have recently shown that presymptomatic Syn I/II/III KO mice display an impaired tonic current, due to defects in GABA release and spillover, leading to diffuse hyperexcitability of hippocampal pyramidal neurons [42] . It is tempting to speculate that the lack of asynchronous inhibitory release in the hippocampus of Syn II mice, by decreasing the tonic inhibition of excitatory neurons, directly contributes to the aberrant network synchronization and epileptogenesis. Animals Experiments were performed on homozygous Syn II KO mice generated by homologous recombination and age-matched C57BL/6J wild-type (WT) animals. All experiments were carried out in accordance with the guidelines established by the European Communities Council (Directive 2010/63/EU of 22 September 2010) and were approved by the Italian Ministry of Health. Preparation of slices After anaesthesia with isoflurane, horizontal hippocampal slices (400 μm thickness) from 3-week-old WT and KO mice were cut using a Microm HM 650 V microtome equipped with a Microm CU 65 cooling unit (Thermo Fisher Scientific, Waltham, MA) at 2 °C in a solution containing (in mM): 87 NaCl, 25 NaHCO 3 , 2.5 KCl, 0.5 CaCl 2 , 7 MgCl 2 , 25 glucose, 75 sucrose and saturated with 95% O 2 and 5% CO 2 . After cutting, we let the slices recover for 30–45 min at 35 °C and for 1 h at room temperature in recording solution. Patch-clamp recordings Whole-cell recordings were performed with a Multiclamp 700B/Digidata1440A system (Molecular Devices, Sunnyvale, CA) on visually identified dentate granule cells using an upright BX51WI microscope (Olympus, Tokyo). We recorded mature dentate granule neurons in which R m <300 MΩ [26] . The extracellular solution used for the recordings contained (mM): 125 NaCl, 25 NaHCO 3 , 25 glucose, 2.5 KCl, 1.25 NaH 2 PO 4 , 2 CaCl 2 and 1 MgCl 2 (bubbled with 95% O 2 –5% CO 2 ). In some experiments, CaCl 2 was replaced with an equimolar concentration of SrCl 2 . For all experiments, we used a high-chloride intracellular solution containing (in mM): 126 KCl, 4 NaCl, 1 MgSO 4 , 0.02 CaCl 2 , 0.1 BAPTA, 15 glucose, 5 HEPES, 3 ATP and 0.1 GTP in which the pH was adjusted to 7.3 with KOH and osmolarity was adjusted to 290 mosmol l −1 with sucrose. Experiments were performed at room temperature apart from a subset of data ( Fig. 6 ) performed at 34 °C. Recordings of evoked and spontaneous inhibitory postsynaptic currents (eIPSCs and sIPSCs) were done at a holding potential ( V h ) of −80 mV in the presence of 50 μM D -APV, 10 μM CNQX, 5 μM CGP 55845 (all from Tocris Bioscience, Ellisville, MO) and of mIPSCs after subsequently adding 0.3 μM TTX (Tocris Bioscience) to the above-mentioned drugs. Evoked excitatory postsynaptic currents were done at a holding potential ( V h ) of −80 mV in the presence of 30 μM bicuculline and 5 μM CGP 55845 (all from Tocris Bioscience, Ellisville, MO) 0.5 μM ω-Agatoxin IVA and 1 μM ω-Conotoxin GVIA (Tocris Bioscience, Ellisville, MO) were used to block P/Q and N-type Ca 2+ channels, respectively. eIPSCs were evoked in granule cells in response to extracellular stimulation of the medial perforant path with a monopolar glass electrode (intensity: 50–150 μA, duration: 30 μs) filled with ACSF and connected with an isolated pulse stimulator (A-M Systems, Carlsborg, WA). The criteria used to define the extracellular stimulation were: (1) no failures in response to repeated 0.1 Hz stimulation; (2) postsynaptic responses at least threefold higher than the square root of noise; (3) latency and shape of synaptic current remained invariant. After finding a cell that met these criteria, we continued all the experiments at stimulation intensity 10% higher than the minimal needed, to avoid possible failures. See Supplementary Methods for additional details on the electrophysiology of primary neuronal cultures Data analysis All data were acquired with Clampex 10.2 and analysed offline with Clampfit 10.2 (pClamp, Molecular Devices, Sunnyvale, CA) and MiniAnalysis (Synaptosoft, Decatur, GA). We inspected eIPSCs visually and considered only those that met the stimulation criteria (see above) and were not contaminated by spontaneous activity. Because of the high intrinsic variability of eIPSCs, 10–30 consecutive responses (at a stimulation frequency of 0.1 Hz) were averaged before the calculation of the peak amplitude and of the kinetic parameters. We considered the peak amplitude as the difference between baseline and the peak of the evoked response; charge as the area under the response; latency as the time from the stimulus artifact to the initiation of a postsynaptic response; rise time as the 10–90% time from the initiation of a response to the peak amplitude; The eIPSC and mIPSC deactivation response was fitted by double exponential equations of the form I ( t )= A fast exp(− t / τ fast )+ A slow exp(− t / τ slow ), where I ( t ) was the amplitude of IPSCs at time t , A fast and A slow were the amplitudes of the fast and slow decay components, respectively, and τ fast and τ slow the corresponding decay time constants. The size of the RRP of synchronous release (RRP syn ) and the probability that any given SV in the RRP will be released ( P ves ) were calculated using the cumulative amplitude analysis [17] , [33] . RRP syn was determined by summing up the peak amplitudes of IPSC responses during a 2-s stimulation train at 40 Hz. The last 40 data points were fitted by linear regression and back-extrapolated to time 0. The intercept with the y axis yielded the RRP syn , and the ratio between the first eIPSC amplitude and RRP syn yielded the P ves . In the same way, we measured RRP tot by calculating the total area of the response induced by each stimulus of the train [17] , [33] , after subtracting the offset to the baseline. We measured the delayed asynchronous release as the 1-s area of the postsynaptic current following a 40 Hz train, normalized to the 1-s area preceding the train (sIPSC area averaged from 5–10 s before the train). This measure of delayed asynchronous release considers both the offset of the last response of the stimulus train to the baseline, as well as the increase in the frequency of the spontaneous postsynaptic currents. To analyse PPD, two brief stimulation pulses were applied at ISIs ranging between 10 and 4,000 ms (10–20 sweeps for each trial). Paired-pulse ratio (PPR) was calculated from the equation: PPR=100 × ( I 2 − I 1 )/ I 1 , where I 1 and I 2 are the mean amplitudes of the eIPSCs evoked by the conditioning and test stimuli, respectively [17] . Analysis of the pre/postsynaptic locus of PPD was performed as described by Malinow and Tsien [32] . We calculated: where CV is the coefficient of variation, A is the peak amplitude of each response and σ is the variance of the peak amplitudes in a series of consecutive responses. From the binomial distribution of transmitter release: because A 2 / σ 2 =( Npvz ) 2 / Np (1− p ) (vz) 2 = Np /(1− p ), where p is the probability of release for each available quanta ( N ), v is the vesicular content and z is the postsynaptic response to a fixed amount of transmitter. On a linear plot ( Fig. 2 ), the depression induced by the second stimulus ( A 2 / A 1 ) with respect to the ratio of coefficients of variation ((CV 2 /CV 1 ) −2 ) should fall under the line if the cause of the depression is presynaptic according to equations (1) and (2) [31] , [32] . Immunoprecipitation Cortical neurons at 10–14 DIV were lysed in RIPA buffer (50 mM Tris–HCl pH 7.4, 150 mM NaCl, 2 mM EDTA, NP40 1%, SDS 0.1%) plus protease inhibitors (complete EDTA-free protease inhibitors, Roche Diagnostic, IN) for 1 h at 4 °C under constant agitation. After centrifugation at 16,000 g for 30 min, protein concentration was quantified with Bradford Protein Assay (BioRad, Segrate, Italy). Protein lysates (1.5 mg per sample) were precleared using 25 μl protein G-Sepharose Fast Flow (GE Healthcare) for 1 h at 4 °C. Precleared lysates were incubated overnight at 4 °C with 5 μg of syn I or syn II antibodies, or anti-HA antibodies as control; immunocomplexes were then isolated by adding either protein G-Sepharose for synII, or anti-mouse IgG-coated Sepharose beads (no. 5946 Cell Signaling) for syn I, for 3 h at 4 °C. SDS–PAGE and western blotting were performed on precast 4–12% NuPAGE Novex Bis-Tris Gels (Life Technologies, Monza, Italy). After incubation with primary antibodies, membranes were incubated with fluorescently-conjugated secondary antibodies (ECL Plex goat α-rabbit IgG-Cy5, ECL Plex goat α-mouse IgG-Cy3) and revealed by a Typhoon TRIO+ Variable Mode Imager (both GE Healthcare, Milano). The following primary antibodies were used: monoclonal anti-Syn I (clone 10.22 [60] ), anti-Syn II (clone 19.21 [60] ) and anti-HA (no. 32-6700 Life Technologies), polyclonal antibodies anti-Cav2.1 (P/Q), anti-Cav2.2 (N) and anti-Cav2.3 (R) (no. C1353, C1478 and C1853, Sigma, Milano, Italy). Statistical analysis All data are presented as mean±s.e.m. with n =neurons/mice. For each group of data, an F -test for the comparison of the variances was used before the statistical testing. In case of non-homogeneity of variance, the statistical analysis was performed using the non-parametric Welch’s t -test for unequal variances. In the case of equal variances, we used the two-tailed unpaired Student’s t -test. Paired t -tests were used according to the experimental design. How to cite this article: Medrihan, L. et al. Synapsin II desynchronizes neurotransmitter release at inhibitory synapses by interacting with presynaptic calcium channels. Nat. Commun. 4:1512 doi: 10.1038/ncomms2515 (2013).